Macroscopic scattering of cracks initiated at single impurity atoms Brittle crystals, such as coloured gems, have long been known to cleave with atomically smooth fracture surfaces, despite being impurity laden, suggesting that isolated atomic impurities do not generally cause cracks to deflect. Whether cracks can ever deviate when hitting an atomic defect, and if so how they can go straight in real brittle crystals, which always contain many such defects, is still an open question. Here we carry out multiscale molecular dynamics simulations and high-resolution experiments on boron-doped silicon, revealing that cracks can be deflected by individual boron atoms. The process, however, requires a characteristic minimum time, which must be less than the time spent by the crack front at the impurity site. Deflection therefore occurs at low crack speeds, leading to surface ridges which intensify when the boron-dopage level is increased, whereas fast-moving cracks are dynamically steered away from being deflected, yielding smooth cleavage surfaces. Chemomechanical problems in which the behaviour of a material is determined by complex interrelated chemical and mechanical processes, such as the interaction between cracks and atomic impurities, are traditionally very hard to investigate both experimentally and theoretically, for a number of reasons. Experimentally, there is a demanding requirement for extremely pure samples, whereas the tight coupling of length scales makes these problems hard to tackle through computer simulation. In this work, we selected boron-doped silicon crystals as optimal systems for investigating these processes, as ultrapure samples are available at graded dopant densities and can be prepared for highly controlled experimental fracture testing [1] , [2] . On the theoretical side, traditionally, fracture mechanic problems have been tackled with continuum mechanics techniques, which have been very successful in predicting many aspects of the failure of brittle single crystals [3] , [4] , [5] , [6] , [7] . However, quantitative predictions of more complex phenomena, for example, the fracture toughness of a material, or how defects such as dislocations scatter cracks [8] , have remained elusive. This is because stress concentration leads to a breakdown of linear elasticity near the crack tip [9] , [10] so that the fracture behaviour depends very strongly on the details of the atomic interactions at the advancing tip, particularly due to the phenomenon known as lattice trapping, whereby the underlying discreteness of the atomic lattice introduces a barrier to crack advancement [11] , [12] . For materials such as silicon, with highly directional covalent bonding, a chemically accurate description of the breaking of bonds at the crack tip requires a quantum mechanical (QM) treatment [13] . QM calculations on small model systems have been used to explain many static aspects of brittle fracture, for example, the directional anisotropy on the Si{110} cleavage plane [7] . However, thousands of atoms contribute significantly to the highly anisotropic stress field driving the crack forward, and must be explicitly represented for accurate simulation of fracture dynamics. These atoms occupy a region far too large to describe with the currently available QM techniques based on density functional theory (DFT). The intrinsically multiscale nature of the fracture problem therefore requires a coupled quantum mechanics/molecular mechanics (QM/MM) approach, which allows both the local chemistry at the crack tip and the large stress gradients near the tip to be represented in a single atomistic model system [14] , [15] , [16] . We carried out our simulations using the Learn on the Fly scheme [17] , which achieves nearly seamless coupling between the quantum and classical parts of the system. This allows a small mobile QM (treated at the DFT level) region tracking the crack tip to be embedded in a much larger interatomic potential region, allowing, for example, impurity-induced stress corrosion phenomena to be investigated [18] . Most previous studies of interactions between cracks and point defects have focused on ductile materials [19] , where long-range elasticity and impurity mobility are more important than the local chemical interactions we focus on here. For example, stress-driven migration of defects towards a crack has been found to have a role in hydrogen-induced embrittlement of metals [20] . However, substitutional boron impurities in silicon are known to be very stable and have very low mobility compared with typical crack speeds, as dopant diffusion typically requires a reaction with a silicon self-interstitial to form a mobile B I complex [21] . Boron clusters and interstitials in the Si matrix have been investigated using both ab initio methods [22] and experiments [23] , but these more complex defects are much rarer than single substitutional atoms. To summarize, although crucial for tuning electronic and vibrational properties [24] , these impurities have only a minimal effect on the mechanical properties of silicon at room temperature. In particular, they do not significantly affect the elastic properties even at rather high dopant concentrations [25] , and they affect plasticity by promoting dislocation mobility at temperatures above the brittle to ductile transition [26] . Whether dopants can influence crack propagation and, namely, scatter an advancing crack from its original cleavage plane is however not clear [6] , [7] . Here we use multiscale molecular dynamics simulations and high-resolution experiments on boron-doped silicon to demonstrate that cracks can be deflected by individual boron atoms. We find that the process requires a characteristic minimum time, which must be less than the overall time spent by the crack front at the B impurity site. We also experimentally observe microscopic deflection in B-doped Si crystals. This involves independent initiation of micron-sized surface ridges, which intensify if we increase the B-dopage level. A simple model shows that if the ridges initiate following crack deflection at B atoms, their spatial distribution along the crack propagation direction must take a universal Rayleigh form. This fits well our experimental observations at 1.10 × 10 19 cm −3 B-dopant concentration, and then correctly predicts the much coarser distribution observed in experiments at 1.05 × 10 15 cm −3 dopant concentration. Taken together, our results show that single substitutional impurities can cause crack deflection in a brittle crystal, contrary to the common assumption. This could be generally true and still consistent with the perfectly smooth fracture surfaces commonly obtained by fast cracking. Indeed, these two facts can be reconciled by the velocity-dependent nature of the crack deflection process, possible only at low speeds, whereas fast-moving cracks are dynamically steered away from being deflected, yielding smooth cleavage. Multiscale QM/MM simulations We first considered fracture in a pure silicon crystal on a low-energy {111} cleavage plane, with the crack propagating in the [211] direction ( Fig. 1a ). As was done in many previous studies [6] , [7] , [14] , [15] , [16] , [17] , [18] , [27] , periodic boundary conditions were used along the crack front direction, a fully three-dimensional investigation being, for now, out of reach of DFT-based atomistic simulations. Previous work [16] has revealed that at speeds below about 1,000 ms −1 , a crack-tip reconstruction consisting of a five- and seven-membered ring related to the π-bonded Pandey 2 × 1 reconstruction of the (111) surface [28] forms spontaneously. Because of the broken mirror symmetry of the crystal with respect to {111} planes, the five–seven crack tip reconstruction can form on only one of the two fracture surfaces [27] , the lower surface with respect to the axes of Fig. 1 , meaning that successive tip reconstruction events can build up to form large-scale surface features via a positive feedback sinking process [16] . We carried out calculations at an increased static loading equivalent to an energy release rate of G 0 =14 Jm −2 , which leads to a stable crack propagation at 1,400 ms −1 ( Fig. 1b and Supplementary Movie 1 ), confirming that at this higher speed the crack is dynamically steered away from forming the reconstructed tip in pure Si. The bond rotation required to form the five–seven crack tip reconstruction would take more time than is sufficient for this faster crack tip to advance by a bond, leaving no chance of it falling into the trap and initiating the sinking behaviour proposed in ref. 16 . 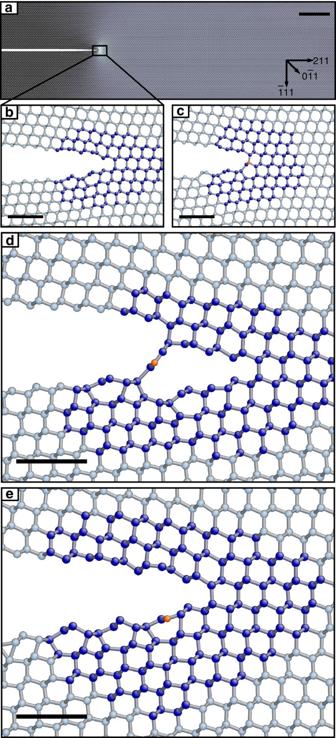Figure 1: Interaction between cracks on Si{111} cleavage planes and B impurities. (a) The multiscale QM/MM simulation system, which has dimensions 1,200 × 400 × 3.84 Å3, and contains around 90,000 atoms. Atoms are coloured by their principal stress eigenvalue, with black corresponding to zero stress and white to high stress. (b) A close-up image of the crack tip showing stable crack propagation in a pure silicon system at 1,400 ms−1(see alsoSupplementary Movie 1). The dark-blue silicon atoms are treated with QM accuracy, and the grey atoms are treated with an interatomic potential. Note the π-bonded 2 × 1 Pandey reconstruction of alternating pentagons and heptagons on the lower fracture surface. (c) Identical system to panelb, but with a single silicon atom replaced by a substitutional boron impurities (orange). When the moving crack encounters a boron impurity, it undergoes a tip reconstruction via a bond rotation and, subsequently, steps down by one atomic layer, (d) (Supplementary Movie 2). At higher speeds, (e), at 1,700 ms−1, the crack passes over the impurity without interacting (Supplementary Movies 3 and 4). Scale bar, 100 Å (ina); scale bar, 10 Å (in all subsequent panels). Figure 1: Interaction between cracks on Si{111} cleavage planes and B impurities. ( a ) The multiscale QM/MM simulation system, which has dimensions 1,200 × 400 × 3.84 Å 3 , and contains around 90,000 atoms. Atoms are coloured by their principal stress eigenvalue, with black corresponding to zero stress and white to high stress. ( b ) A close-up image of the crack tip showing stable crack propagation in a pure silicon system at 1,400 ms −1 (see also Supplementary Movie 1 ). The dark-blue silicon atoms are treated with QM accuracy, and the grey atoms are treated with an interatomic potential. Note the π-bonded 2 × 1 Pandey reconstruction of alternating pentagons and heptagons on the lower fracture surface. ( c ) Identical system to panel b , but with a single silicon atom replaced by a substitutional boron impurities (orange). When the moving crack encounters a boron impurity, it undergoes a tip reconstruction via a bond rotation and, subsequently, steps down by one atomic layer, ( d ) ( Supplementary Movie 2 ). At higher speeds, ( e ), at 1,700 ms −1 , the crack passes over the impurity without interacting ( Supplementary Movies 3 and 4 ). Scale bar, 100 Å (in a ); scale bar, 10 Å (in all subsequent panels). Full size image However, if a substitutional boron impurity is placed in the path of the crack, we find that a chemical interaction with the passing crack leads to a new five–seven tip reconstruction located at the defect site ( Fig. 1c and Supplementary Movie 2 ). The boron atom readily forms sp 2 bonds with three neighbouring silicon atoms at a bond angle of 120°. This significantly stabilizes π-bonded chains, promoting the subsequent formation of linear chains ( Fig. 1d ), eventually leading to the crack slowing and stepping down by one atomic plane in the [ ] direction. We note that the lack of mirror symmetry between the upper and lower fracture surfaces and the 2 × 1 fracture surface reconstruction geometry imply that an advancing fracture can encounter B atoms located at four inequivalent sites. We carried out simulations for all these cases and found that stepping occurs only for B atoms located on the lower surface within a seven-membered ring, suggesting that only one out of four of the dopant atoms can yield a crack deflection. When the applied load is further increased to G 0 =18 Jm −2 , the crack speed increases to ~ 1,700 ms −1 . At this speed, we find there is no longer sufficient time for bond rotation and π-bonded structure formation to occur before the crack moves on to the next bond, and the crack passes straight through any boron impurity site ( Fig. 1e , Supplementary Movies 3 and 4 ). To summarize, our DFT calculations suggest that at speeds below ~ 1,500 ms −1 , crack deflection caused by individual B atoms can be observed at a rate determined by B concentration, whereas perfectly smooth fracture surfaces should be obtained in B-doped samples above this speed. We note that a speed-hindered crack deflection scenario could help rationalize how mirror smooth cleavage can be obtained in many brittle specimens, regardless of their impurity concentration, as long as fast cracking is ensured. Fracture experiments We carried out experiments on the fracture behaviour in boron-doped silicon in a three-point bending (3PB) loading geometry at two different dopant concentrations, details of which are presented in Table 1 . In the 3PB technique, the crack front advances as a quarter ellipse (schematically illustrated in Fig. 3a , with the driving force for crack propagation and, hence, the crack velocity, decreasing from the bottom of the specimen to the top (see Methods, and ref. 29 ). A wide range of crack velocities can thus be obtained in a single experiment. Micrographs of the fracture surfaces obtained at low- and high dopant concentrations are shown in Fig. 2a,b . At high speeds (bottom of each image), the fracture surface is atomically smooth, but as the velocity decreases below a critical value of around 1,200 ms −1 , micrometre-scale ridges develop out of the fracture plane (that is, in the [ ] direction), and with the ridge spines pointing along the [211] direction, aligned with the white arrows in Fig. 2a,b . These ridges are similar in shape to those observed during low-speed cracking of Si samples in a previous work [16] . Table 1 Features of the observed ridge patterns. 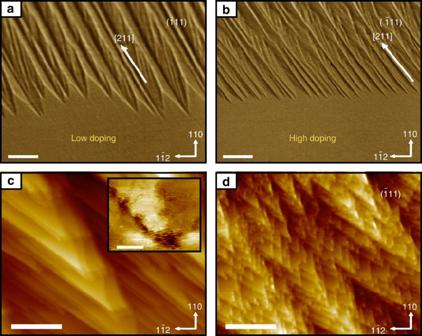Figure 2:Observations of ridge development on Si{111} cleavage planes below a critical velocity. In the 3PB experimental loading geometry, crack velocity deceases moving up the figure. Confocal microscopy images of the ridge patterns observed inpost-mortemanalysis of the fracture surfaces in samples containing (a) low dopant concentration of 1.05 × 1015cm−3and (b) high dopant concentration of 1.10 × 1019cm−3. Scale bar, 20 μm. Ridges always form in the out-of-planedirection and along the [211] direction as indicated by the white arrows. The low-doping sample has larger lateral ridge spacing along the crack front, and increased roughness perpendicular to the crack front. (c,d) STM close-ups (scale bar, 1 μm) of thein situfracture surface for both doping levels. At high doping levels, there are many more submicron scale ridges that do not go on to form macroscopic surface features. Inset, an STM close-up showing a single ridge initiating at a well-defined nanometre-scale point (scale bar, 20 nm). Full size table Figure 2: Observations of ridge development on Si{111} cleavage planes below a critical velocity . In the 3PB experimental loading geometry, crack velocity deceases moving up the figure. Confocal microscopy images of the ridge patterns observed in post-mortem analysis of the fracture surfaces in samples containing ( a ) low dopant concentration of 1.05 × 10 15 cm −3 and ( b ) high dopant concentration of 1.10 × 10 19 cm −3 . Scale bar, 20 μm. Ridges always form in the out-of-plane direction and along the [211] direction as indicated by the white arrows. The low-doping sample has larger lateral ridge spacing along the crack front, and increased roughness perpendicular to the crack front. ( c , d ) STM close-ups (scale bar, 1 μm) of the in situ fracture surface for both doping levels. At high doping levels, there are many more submicron scale ridges that do not go on to form macroscopic surface features. Inset, an STM close-up showing a single ridge initiating at a well-defined nanometre-scale point (scale bar, 20 nm). Full size image The data in Table 1 show that at higher dopant concentrations, independent ridge initiation events occur much closer to a unique common height in the sample, or equivalently within a smaller velocity interval during crack front deceleration, leading to a much smoother microscale ridge front ( Fig. 2b ). The lateral spacing of the ridges d , however, is only slightly affected, as the ridges are in both cases well spaced, with lateral spacings always of the order of 10 μm, which is much larger than the average distance of 4.5 nm between B dopants at the highest doping level investigated here. This indicates that although B atoms promote ridge initiation, some selection must be taking place during initiation and growth from the nanometre to the micrometre scale, yielding the observed lateral micrometre-scale spacing illustrated in Fig. 2a,b . A likely seed for well-spaced micrometre-scale ridges is the generation and bunching of misalignment steps known to take place on the vicinal Si{111} surfaces [30] , which result from extremely small but inevitable misalignments of the sample in the loading jig [2] . However, and irrespective of the growth selection mechanism, we note that if the ridges were to initiate following crack deflection at individual B atoms in crack front sections free from misalignments steps, as suggested by our simulations, many much smaller ridges would have to be found on the cleavage surface, that is, those ridges which initiated anywhere the crack front speed was appropriately low, but did not eventually grow. Such ridges do exist as revealed by close-up scanning tunnelling microscopy (STM) images such as those reported in Fig. 2c,d , which show that there are many nanometre-scale ridges within each micrometre-scale one, and indicate that the nanoscale ridges initiate at well-defined points ( Fig. 2c , inset). We next note that although the ridge growth selection process is likely to be significantly complex, there will be simple properties that the micrometre-scale ridge distribution strictly must possess if the individual nanometre-scale ridges result from causally independent scattering events originated at individual B atoms. In particular, the distribution of the positions where the ridges initiate measured along the crack propagation direction will depend on B concentration, for example, it will necessarily get broader if the B concentration is sharply decreased, consistent with our observations. The s.d. R of such a distribution can be visualized as the roughness of the boundary between the smooth and ridged regions of our fracture surfaces (shown with the red and blue lines in Fig. 3b–e ). To explore these ideas, we further analyse the propagating crack front, as it decelerates advancing through the specimen and forms a pattern of ridges similar to that illustrated schematically in Fig. 3a . We assume that the ridge tips pinpoint events independent from each other, which is possible under appropriate conditions met by our systems ( cf. Supplementary Note 1 ). The distribution of these events along the crack propagation direction will thus simply reflect the statistics of where deflection occurs for a crack front point progressing on a cleavage plane containing randomly distributed boron impurities of known average density. This allows us to construct a simple one-dimensional model, described below, for the single crack scattering event, based on the hypothesis that within the interval of speeds relevant for ridge initiation crack deflection can follow each B encounter event with a velocity-dependent probability. 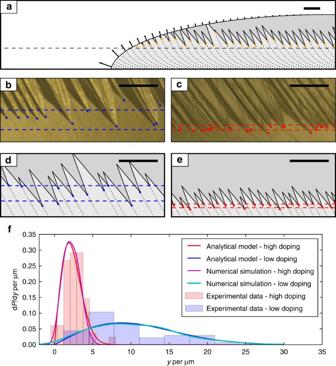Figure 3: Model for the initiation of ridge features on the fracture surface. (a) Schematic showing dynamics of ridge formation. The elliptical crack front propagates from right to left, starting at the bottom right-hand corner with the normal crack front velocity, shown by the black arrows, decreasing from the bottom to the top of the specimen. Ridges form with a velocity-dependent probability, which increases as the velocity decreases below a critical velocityVc~ 1,200 ms−1(the black dashed line corresponds to this velocity). The ridges originate independently along the black dotted lines, which represent step-bunched regions of the vicinal Si () surface. Scale bar, 100 μm. Ridge profiles observed in the experiment (b,c) and predicted by the model (d,e) for low doping (b,d; concentration 1.05 × 1015cm−3) and high doping (c,e; concentration 1.10 × 1019cm−3) cases. The blue and red dashed lines represent the roughness of the vertical ridge initiation positions, and are drawn at one s.d. above and below the mean. Scale bar, 20 μm for these four panels. (f) Comparison of ridge initiation model with experimental data. The red and blue solid curves show the probability distribution of ridge initiation as a function of vertical distance, as predicted by the one-dimensional model described in the text, and the histograms are the same data measured from confocal microscopy images of fracture specimens at two different doping levels. The magenta and cyan curves show the distributions obtained in the more detailed two-dimensional numerical simulations illustrated indande. Figure 3: Model for the initiation of ridge features on the fracture surface. ( a ) Schematic showing dynamics of ridge formation. The elliptical crack front propagates from right to left, starting at the bottom right-hand corner with the normal crack front velocity, shown by the black arrows, decreasing from the bottom to the top of the specimen. Ridges form with a velocity-dependent probability, which increases as the velocity decreases below a critical velocity V c ~ 1,200 ms −1 (the black dashed line corresponds to this velocity). The ridges originate independently along the black dotted lines, which represent step-bunched regions of the vicinal Si ( ) surface. Scale bar, 100 μm. Ridge profiles observed in the experiment ( b , c ) and predicted by the model ( d , e ) for low doping ( b , d ; concentration 1.05 × 10 15 cm −3 ) and high doping ( c , e ; concentration 1.10 × 10 19 cm −3 ) cases. The blue and red dashed lines represent the roughness of the vertical ridge initiation positions, and are drawn at one s.d. above and below the mean. Scale bar, 20 μm for these four panels. ( f ) Comparison of ridge initiation model with experimental data. The red and blue solid curves show the probability distribution of ridge initiation as a function of vertical distance, as predicted by the one-dimensional model described in the text, and the histograms are the same data measured from confocal microscopy images of fracture specimens at two different doping levels. The magenta and cyan curves show the distributions obtained in the more detailed two-dimensional numerical simulations illustrated in d and e . Full size image Ridge initiation model Our QM calculations suggest that there are two independent time scales that are important to determine the ridge-initiation probability. These are defined by the time for the crack to advance by one bond, set by the crack velocity and the spacing between bonds, and by the time necessary for the process inducing the deflection to occur, as observed in our simulations. The latter time will be furthermore blurred by the (shorter) period Δ T of the oscillation that triggers the deflection process, which will be at best in phase and at worst in anti-phase at the time of crack front arrival. To derive the model, described in more detail in Supplementary Note 1 , we thus assume that the B-induced tip reconstruction event necessary for ridge initiation requires a minimum time T c to occur since crack front arrival, and is certain to have happened after a time T c +Δ T if the crack has still not moved on to the next bond. For the velocity range of interest in the current experiments, we make the simple assumptions that the probability for this event rises linearly as a function of time between these two limits, and that there is a fixed probability that a microscopic ridge will grow provided that the event takes place. The resulting ridge initiation probability is zero as long as the crack velocity exceeds some upper critical value V c , and starts increasing as the velocity decreases below it (illustrated schematically in Supplementary Fig. S1 ). Assuming that the deceleration of the crack as it moves through the specimen is approximately constant yields a ridge initiation probability that grows linearly along the propagation axis beyond the critical point, where crack-deflecting interactions are first able to occur. This model is analytically solvable and leads to a Rayleigh distribution for the positions of the ridge initiation points, with a probability density function where the length scale parameter σ is given by the model parameters entering σ , besides Δ T and V c , are the effective dopant concentration n ′, the Si bond spacing a in the propagation direction, the crack deceleration g and the likelihood α that a microscopic ridge will grow after a B-induced crack deflection event, which is simply assumed to be the same at all doping levels and for all ridges, independent of their position and detailed shape. All these parameters, except α , can be found directly from our experimental setup and calculation results, as described in the Methods section, and are given in Table 2 . Notably, the s.d. of the distribution turns out to be inversely proportional to the square root of the linear dopant concentration: this implies that increasing the B linear concentration by a factor of ~ 20 will lead to about a fourfold decrease in the observed roughness. Table 2 Parameters of the ridge initiation model. Full size table We first determine the growth likelihood parameter that best fits the experimental data at 1.10 × 10 19 cm −3 dopant concentration, which fixes it to α =0.12, a value smaller than 1 as expected. The theoretical and experimental ridge initiation distributions corresponding to this high dopage case are illustrated by the red curve and histogram in Fig. 3f , corresponding to the systems shown in Fig. 3c,e . A much broader distribution of ridge initiation points is then predicted by varying n ′ to the value corresponding to the 1.05 × 10 15 cm −3 low-dopant experimental concentration of the system of Fig. 3b,d . This is found to reproduce well the experimental results (blue curve and histogram in Fig. 3f ), indicating that ridge initiation statistics follow the density of B impurities in the expected way. The roughness values produced by the model and observed in the experiments are included in Table 1 . A more detailed model fully representing the space-dependent deceleration of the elliptical crack front was also built, and was found to give equivalent results despite introducing a deviation from linearity of the ridge initiation probability as a function of the vertical position coordinate in the specimen ( cf . Supplementary Figs S2 and S3 , and Supplementary Note 1 ). The good agreement between the model and the experiment for the dependence of the ridge patterns on B concentration strongly supports the fact that the surface perturbations seen here do originate at individual B atoms, indicating that an isolated substitutional atom is all that is needed in this system to deflect a crack front approaching at well over 1,000 ms −1 . This is novel with respect to previous work [16] , where details of the initiation of the roughening instability were unknown. Our results identify a possibly general mechanism for the abrupt smooth-to-rough transition of surface morphology often observed in crack deceleration experiments, as this is the behaviour generally predicted by the velocity-dependent mechanism even if the impurity defects responsible for it are uniformly distributed throughout the specimens. In particular, given its simplicity, we expect our rate equation-based model to apply to other systems in which crack propagation interacts with isolated point defects: this could, for example, allow the impurity species responsible for crack deflection to be identified from comparative testing of specimens where the relative concentrations of impurities are varied. Conversely, the existence of a minimum critical time for the atomistic crack deflection initiation processes to take place could provide a natural and economic rationalization for the occurrence of smooth cleavage surfaces in many real materials. This might, for example, apply to impurity-laden crystalline manufactured goods, for which ensuring fast fracturing is traditionally a key processing rule, and yields the prediction of similar behaviour being possible in further materials where observations are currently missing. All that is required is that the crack speed be sufficiently high to hinder all available deflection mechanisms, with no need to try to explain why deflection mechanisms do not exist, or to ensure that they cannot operate in different fracturing conditions. Furthermore, our results suggest that 3PB experiments on intrinsic specimens could be used to identify the minimum speed for smooth cleavage during brittle fracture propagation, and that substitutional impurity content is one of the factors controlling the roughness of cleavage surfaces and, as such, should be taken into account when operatively defining the fracture toughness of crystalline specimens. At a more practical level, crystalline surface samples hosting asperities with finely controlled slope, height and spacing could be useful in experiments carried out to calibrate adhesion/friction models [31] , [32] , or to tune the interfacial properties that govern boundary and mixed lubrication in tribological applications in MEMS [33] . Multiscale QM/MM simulations The Learn on the Fly hybrid simulations illustrated in Fig. 1 were carried out using the libAtoms/QUIP code [34] , which combines (i) the Stillinger–Weber (SW) classical interatomic potential [35] that captures long-range elastic relaxation and (ii) a QM model based on DFT, as implemented in the CASTEP [36] and VASP [37] packages, to describe the crack tip region where bond-breaking takes place. For the DFT calculations, ultrasoft pseudopotentials [38] and the PW91 generalized gradient approximation to the exchange correlation functional were used [39] . A planewave basis set with a cutoff energy of 250 eV and a Monkhorst–Pack mesh with 1 × 1 × 4 k -points were used. The crack tip region contained around 100 QM atoms, to which a hysteretic buffer region of 7–9 Å was added to give accurate forces [40] , leading to QM atom-buffered clusters containing 200–300 atoms. Each force calculation took around 5–10 min on 64 cores on a standard commodity cluster. The SW interatomic potential [35] was used to describe atoms away from the crack tip, after adjustment to match the lattice constant and bulk modulus of the QM models. Note that we used the original SW parameterization, and not the modified version [41] , which was made brittle by increasing the strength of the three-body term: treating the bond-breaking processes at the crack tip region at the DFT level removes the need to modify the potential parameters to obtain brittle behaviour. Constant temperature (300 K) simulations were carried out on a 1,200 × 400 × 3.84-Å 3 slab containing 90,868 atoms. Note that the [211] × [ ] × [ ] crack system presented here is equivalent to the [ ] × [111] × [ ] system of our earlier work [16] because of the 120° rotational symmetry about the {111} axis, which is a property of the Fd m spacegroup. The system was equilibrated by propagating a crack from rest at a load of G 0 =14 Jm −2 , which, after 10 ps of equilibration, leads to a stable crack propagation at a velocity of 1,400 ms −1 , with the velocity remaining constant within about 50 ms −1 throughout the 5–10 nm of further propagation along which we investigate crack scattering. The boron substitutional impurities were always introduced at least 20 Å ahead of the moving crack tip to allow time for equilibration. The higher-speed system shown in Fig. 1e was obtained by rescaling a snapshot from the 1,400 ms −1 simulation to a load of G 0 =18 Jm −2 and re-equilibrating until fluctuations in the crack velocity were again less than 50 ms −1 . The simulations were carried out with a slab thickness of 3.84 Å, with periodic boundary conditions along the crack front. This value ensures that all the nearest neighbours of the B impurities are silicon atoms, so that there are no boron chains in our model system. As the relevant chemical effects are of local character, we do not expect any qualitative changes to our results if a deeper simulation cell were used; however, we cannot completely exclude the possibility of spurious effects arising from the use of periodic boundary conditions. Simulation movies are available online as Supplementary Movies 1–4 . Fracture experiments Cleavage of 525- (low doping) and 381-μm (high doping) thick boron-doped silicon specimens of lateral dimensions 43 × 15 mm and boron dopant concentrations of 1.05 × 10 15 cm −3 and 1.10 × 10 19 cm −3 was performed under 3PB. The specimens were notched with a 150-μm thick diamond saw to a length of around 0.15 mm (ref. 2 ). With reference to the geometry of Figs 2 and 3 , the crack initiates at the bottom right corner of the specimen and starts to propagate as a quarter circular crack, becoming elliptical while reaching the steady state, as illustrated in Supplementary Fig. S4a,b . A wide range of crack normal speeds V n are obtained along the curved crack front, from thousands of ms −1 at the bottom surface to several tens of ms −1 at the top. It has been previously shown [29] that the advancing crack front can be accurately modelled by an ellipse with major axis a =3 h and minor axis b =0.8 h , where h is the height of the specimen, as shown in Supplementary Fig. S4c . We calculated the velocity and acceleration of a point P on the elliptical crack front by considering the motion of the osculating circle to the ellipse at P , defined to be the circle with common normal and radius of curvature to the ellipse at P , shown with a dashed line in Supplementary Fig. S4c . The radius r of the osculating circle and the angle θ between the x axis and the crack front normal at P can be determined purely geometrically, and are functions of the y coordinate of P . For an elliptical front advancing at a constant speed V x , the crack front normal velocity is simply the component of V x in the normal direction, V x cos θ , and the point P can be seen to undergo circular motion in the osculating circle of radius r with tangential velocity V t = V x sin θ , with an effective centripetal acceleration a n of magnitude V t 2 / r . Plots of the calculated values of θ , V n and a n as functions of y are given in Supplementary Fig. S5 for an example specimen where V x =2,200 ms −1 , specimen height h =515 μm and ellipse axes are a =3 h and b =0.8 h . In our experimental studies, x is aligned with the [ ] direction and y with the [110] direction. We find that corrugated ridges start to form at y / h =1/3, when the normal to the crack front is at an angle close to θ =60° to the x direction and the crack is propagating close to the crystallographically favourable [211] direction. Our QM/MM computer simulations correspond to fracture propagation along this [211] line. For the example illustrated with the dashed lines in Supplementary Fig. S5 , at a vertical position of y c =170 μm, the normal crack velocity is V n =1,100 ms −1 and the normal acceleration is a n =−5.5 × 10 9 ms −2 . The critical crack normal velocity V n below which ridge initiation is possible is inferred from measurements of V x and the average height y in the sample at which the ridges initiate, using the known dynamics of the 3PB crack front outlined above. The notch length determines the crack velocity V x at a steady state, which, in this case, was around 2,200 ms −1 , measured using a potential drop technique [42] , [2] . We estimate the uncertainty in V x to be about 100 ms −1 , with a corresponding uncertainty of 50 ms −1 in V n ( y ). We then measured the average vertical height y at which the larger ridges start to develop, using optical microscopy. The absolute uncertainty in this measurement is lower than 10 μm, which for the typical speeds and decelerations given above yields a further contribution to the uncertainty in the normal crack velocity estimated as 60 ms −1 . Combining these two independent sources of error leads to an overall experimental uncertainty in the critical crack normal velocity for the onset of instabilities of around 80 ms −1 . The STM/scanning tunnelling spectroscopy measurements were performed in a variable temperature STM Omicron system under a vacuum of 4 × 10 −11 torr. An electrochemically prepared W tip conditioned by in situ electron bombardment was used for the measurements. Topography images were obtained by applying a bias voltage of 1.2–1.4 V to the sample, and at a tunnelling current set point of 0.5 nA. A feedback loop was adjusted to maintain constant current. Model parameterization To compare the experimentally measured roughness with the predictions of the model described above and derived fully in Supplementary Note 1 , we need to estimate the values of the parameters, which make up the constant σ in equation 2. The spacing between pairs of vertically aligned bonds in the direction of crack propagation, a , can be easily measured from our simulations to be 4.0 Å. The critical ridge initiation speed V c is taken from experimental measurements as discussed above. Similarily, the crack front deceleration g can be approximated using the analysis of the 3PB dynamics outlined above as g = V t 2 /r =( V x sinθ) 2 / r . In pure silicon, the fastest phonon mode has a frequency of 15 THz, which corresponds to a period of Δ T ~ 60 fs. The lower mass of boron results in higher frequency modes (period 55 fs) localized near dopants, but even at the highest doping levels considered here these modes are 50 times less intense than the pure silicon modes [43] . Finally, as our simulations show that only one out of every four boron atoms leads to crack deflection, the effective linear dopant concentrations n ′ are reduced by a factor of four. All these values are reported in Table 2 . We fit the model to the longitudinal positions of the ridge initiation points measured in several highly doped experimental specimens by adjusting the parameter α . Note that as α is a probability, its value is constrained to lie in the range 0≤ α ≤1, with any fitted values outside that range invalidating the model. The fit yields a likelihood of around 12% for a ridge formed along any straight line to grow large enough to become macroscopically observable, which is <1 as required and is consistent with the STM observations of many small ridges in Fig. 2d . We were then able to correctly predict the distribution of ridges found in the low-doping samples without any additional fitting. How to cite this article: Kermode, J. R. et al. Macroscopic scattering of cracks initiated at single impurity atoms. Nat. Commun. 4:2441 doi: 10.1038/ncomms3441 (2013).